Photosynthetic growth despite a broken Q-cycle Central in respiration or photosynthesis, the cytochrome bc 1 and b 6 f complexes are regarded as functionally similar quinol oxidoreductases. They both catalyse a redox loop, the Q-cycle, which couples electron and proton transfer. This loop involves a bifurcated electron transfer step considered as being mechanistically mandatory, making the Q-cycle indispensable for growth. Attempts to falsify this paradigm in the case of cytochrome bc 1 have failed. The rapid proteolytic degradation of b 6 f complexes bearing mutations aimed at hindering the Q-cycle has precluded so far the experimental assessment of this model in the photosynthetic chain. Here we combine mutations in Chlamydomonas that inactivate the redox loop but preserve high accumulation levels of b 6 f complexes. The oxidoreductase activity of these crippled complexes is sufficient to sustain photosynthetic growth, which demonstrates that the Q-cycle is dispensable for oxygenic photosynthesis. Cytochrome b 6 f and bc 1 are homologous protein complexes having a major role in photosynthetic and respiratory electron transport chains. 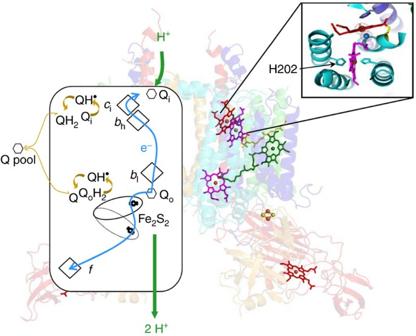Figure 1: The cytochromeb6fdimer operates through a modified Q-cycle. Left, box schematic; theb6fcomplex transfers two protons (green arrows) per electron transferred (blue arrows) along high (Fe2S2cluster, cytochromef) and low potential chains (bl,bh,cihaems). Quinol (QH2) oxidation at Qosite, Quinone (Q) reduction at Qisite. Right, structure (redrawn from ref.35) depicting haemsb(purple),ciand f (red), Fe2S2cluster (yellow and orange ball-and-stick model), cytochromeb6(cyan), subunit IV (blue), Rieske subunit (yellow), cytochromef(red), PetG, L, M and N subunits (green). Magnification of Qisite comprisingbhandcihaems. They contribute to building up the proton motive force via the Q-cycle [1] , [2] depicted in Figure 1 and Supplementary Figure S1 . This redox loop couples the consecutive oxidation of two quinols at the Q o site to the reduction of one quinone at the Q i site through the low-potential chain and of two plastocyanins along the high-potential chain. It increases the ratio of H + pumped per electron transferred and thus the overall energetic efficiency of the complex. In cytochrome b 6 f , the low-potential chain involves two b haems, b l and b h (the subscripts l and h stand for low and high midpoint potential), and a single covalently bound c -type haem, c i [3] , [4] , [5] , [6] , [7] , [8] , in close vicinity with the b h haem as depicted in Figure 1 . In the conditions tested so far, the inactivation of the Q i site of the cytochrome bc 1 of purple photosynthetic bacteria forbids photosynthetic growth [9] , [10] , [11] . In the oxygenic photosynthetic chain, attempts to inactivate the Q-cycle by knocking out the b h haem with mutation of its histidine axial ligand have failed until now because, at variance with the bc 1 case [9] , mutation of His202 dramatically decreases the accumulation of the b 6 f complex [12] . Figure 1: The cytochrome b 6 f dimer operates through a modified Q-cycle. Left, box schematic; the b 6 f complex transfers two protons (green arrows) per electron transferred (blue arrows) along high (Fe 2 S 2 cluster, cytochrome f ) and low potential chains ( b l , bh , c i haems). Quinol (QH 2 ) oxidation at Q o site, Quinone (Q) reduction at Q i site. Right, structure (redrawn from ref. 35 ) depicting haems b (purple), c i and f (red), Fe 2 S 2 cluster (yellow and orange ball-and-stick model), cytochrome b 6 (cyan), subunit IV (blue), Rieske subunit (yellow), cytochrome f (red), PetG, L, M and N subunits (green). Magnification of Q i site comprising b h and c i haems. Full size image Here we engineered in the green alga Chlamydomonas reinhardtii a strain restoring the accumulation of b 6 f complexes although lacking haems b h and c i . We show that it sustains photosynthetic growth and propose a mechanism accounting for this growth despite a broken Q-cycle. The Q i KO strain has b 6 f complexes but lacks haems b h and c i To overcome the accumulation defect resulting from the H202Q mutation in the petB gene encoding cytochrome b 6 , we genetically combined it with the R420C mutation [13] , [14] in the chloroplast protease FtsH1. The double mutant, referred to as Q i KO , contains a wild-type level of cytochrome b 6 f complex ( Fig. 2a,b ), which is in marked contrast with the parental single mutant petB-H202Q . 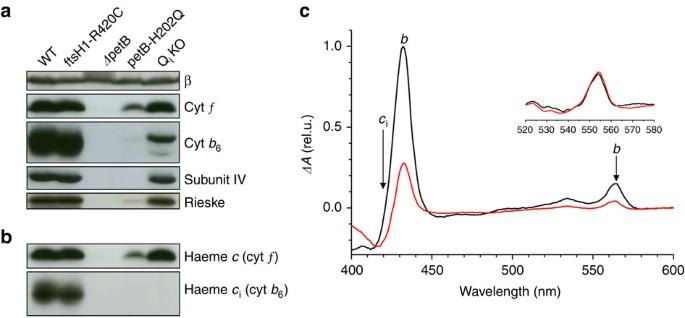Figure 2: Characterization of cytochromeb6fcomplex in theQiKOstrain. (a) Immunoblot chemiluminescence analysis of the major subunits of cytochromeb6f. Subunit β of chloroplast ATPase as a loading control.QiKOshows wild-type level of all cytochromeb6fsubunits with the doublet signature for cytochromeb6missing thecihaem after SDS-urea PAGE. (b) Covalent haem peroxidasic activity confirms the absence of thecihaem inQiKOstrain. (c) Dithionite minus ascorbate spectra from purifiedb6fcomplexes. Black, WT; red, QiKO. Haemsb(peaks at 434 and 564 nm) andci(broad band at 425 nm) components36; in QiKO the decreased amplitude at 434 and 564 nm demonstrates the absence ofbhand the trough at 420 nm the absence ofci. The spectra have been normalized to the cytochromefcontent (inset). We purified by affinity chromatography [5] the Q i KO b 6 f complex, which contains, expectedly, a decreased amount of b haem (30%) as shown by the UV–visible spectra in Figure 2c . This lower-than-expected content (30 versus 50%) stems from the instability of the solubilized complex. Indeed, we assessed the amount of remaining b haem in vivo and found that it matched the amount of b l haem from the control strain ( Fig. 3a , black filled symbols). Importantly, in addition to lacking the b h haem, the rescued b 6 f complex also lacked the c i haem as evidenced by Figure 2b,c, as suggested for petB-H202Q [6] . We thus successfully recovered, in the Q i KO strain, a b 6 f complex with a fully inactivated Q i site without affecting the other cofactors. Figure 2: Characterization of cytochrome b 6 f complex in the Q i KO strain. ( a ) Immunoblot chemiluminescence analysis of the major subunits of cytochrome b 6 f . Subunit β of chloroplast ATPase as a loading control. Q i KO shows wild-type level of all cytochrome b 6 f subunits with the doublet signature for cytochrome b 6 missing the c i haem after SDS-urea PAGE. ( b ) Covalent haem peroxidasic activity confirms the absence of the c i haem in Q i KO strain. ( c ) Dithionite minus ascorbate spectra from purified b 6 f complexes. Black, WT; red, Q i KO. Haems b (peaks at 434 and 564 nm) and c i (broad band at 425 nm) components [36] ; in Q i KO the decreased amplitude at 434 and 564 nm demonstrates the absence of b h and the trough at 420 nm the absence of c i . The spectra have been normalized to the cytochrome f content (inset). 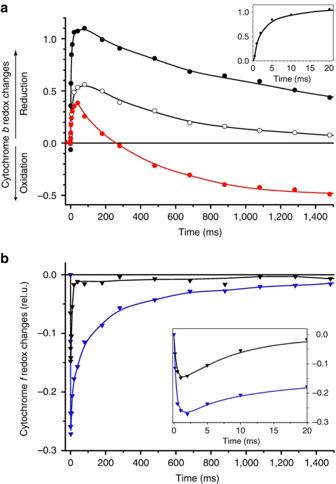Figure 3: Probing electron transferin vivo. (a) Light-induced redox changes of cytochromebinQiKO. Black, filled symbols, mildly reducing conditions; open symbols, after pre-illumination to get similar contents of pre-reduced and pre-oxidized haemb; red, strongly reducing conditions. Inset: reduction component on a smaller time scale. (b) Light-induced redox changes of cytochromefin strongly reducing conditions. Black,WT; blue,QiKO, normalized on the photosystem I amount. Re-reduction of cytochromefinQiKOis rate-limited by the re-oxidation of theblhaem. The reduction of cytochromefinQiKOis biphasic, with the fast component being similar to the WT one (t1/2∼3 ms) (see inset), and the slow component being concomitant with the oxidation ofbl(t1/2∼250 ms). Full size image Figure 3: Probing electron transfer in vivo . ( a ) Light-induced redox changes of cytochrome b in Q i KO . Black, filled symbols, mildly reducing conditions; open symbols, after pre-illumination to get similar contents of pre-reduced and pre-oxidized haem b ; red, strongly reducing conditions. Inset: reduction component on a smaller time scale. ( b ) Light-induced redox changes of cytochrome f in strongly reducing conditions. Black, WT ; blue, QiKO , normalized on the photosystem I amount. Re-reduction of cytochrome f in QiKO is rate-limited by the re-oxidation of the b l haem. The reduction of cytochrome f in QiKO is biphasic, with the fast component being similar to the WT one ( t 1/2 ∼ 3 ms) (see inset), and the slow component being concomitant with the oxidation of b l ( t 1/2 ∼ 250 ms). Full size image Q i KO has a disabled Q i site but retains a wild-type Q o site This was further demonstrated by the functional characterization of the cytochrome b 6 f variant in vivo . The oxidation kinetics of cytochrome f was identical to the wild-type one ( Supplementary Fig. S2 ). Figure 3a shows the transient absorbance changes associated with the redox changes of the b haem. Under mildly reducing conditions ( Fig. 3a , black trace and inset), the reduction of a b haem is similar to that of the wild type, with a half-time of ∼ 2 ms (ref. 15 ). Thus, the Q o site is not impaired. However, contrary to the wild-type case ( Fig. 4 , green trace), this reduction is not electrogenic ( Fig. 4 , black trace), showing that the reduced b haem is on the lumenal side of the membrane and that, as a corollary, the b h haem and the Q i site are indeed knocked out. The Q i KO b 6 f complex is thus genuinely the long-sought variant, inactivated in its Q i site yet retaining a wild type like Q o site, required to assess the dispensable character of the Q-cycle in the photosynthetic chain. 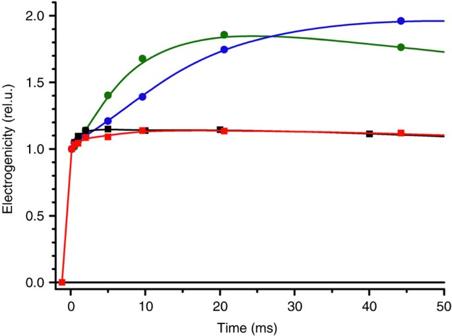Figure 4: Light-induced electrogenicity inQiKOandWT(520–546 nm). QiKO(squares) andWT(circles), black and green, mildly reducing conditions; red and blue, strongly reducing conditions. Figure 4: Light-induced electrogenicity in Q i KO and WT (520–546 nm). Q i KO (squares) and WT (circles), black and green, mildly reducing conditions; red and blue, strongly reducing conditions. Full size image QiKO sustains phototrophic growth In vitro assay (reduction of plastocyanin in the presence of excess plastoquinol [16] ) showed that the Q i KO b 6 f complex sustains a notable electron-transfer flux. The turnover rate is, taking into account that only 30% of b haem is present, 20±4 s −1 , 5% that of wild type (WT) [15] . Although faint, this flux proved to be vital in essence. Indeed, it sustained photosynthetic growth ( Fig. 5 and Supplementary Fig. S3 ). 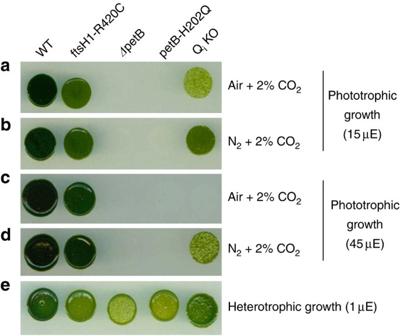Figure 5: Remaining electron flow inQiKOdevoid of Q-cycle sustains phototrophic growth with light enhanced oxygen sensitivity. Cells were plated on minimal medium and grown for 10 days under 15 (a,b) or 45 (c,d) μE m−2s−1of light and a controlled atmosphere combining 2% CO2and 98% air (a,c) and or 98% N2(b,d) to test phototrophic growth. (e) Cells were plated on acetate medium as heterotrophic growth control at very low light fluences (1 μE m−2s−1). Figure 5 shows growth efficiencies under moderate illumination, in the presence (a) and absence (b) of oxygen. As expected from the block in the photosynthetic electron-transfer chain, a b 6 f -lacking mutant showed no phototrophic growth under either condition. This was in contrast to the Q i KO strain, which grew moderately but markedly under phototrophic conditions ( Fig. 5 ). Although this phototrophic growth is oxygen sensitive, the b 6 f -lacking and Q i KO strains grew at a rate similar to that of the wild type in the presence of oxygen, which allows mitochondrial respiration, under heterotrophic conditions (acetate) ( Fig. 5e ). Oxygen per se is thus not detrimental, but the combination of light and oxygen is ( Fig. 5c ), suggesting that photosynthetic activity over-produces reactive oxygen species in the Q i KO strain, as found in the H212N bc 1 case [11] . Figure 5: Remaining electron flow in Q i KO devoid of Q-cycle sustains phototrophic growth with light enhanced oxygen sensitivity. Cells were plated on minimal medium and grown for 10 days under 15 ( a , b ) or 45 ( c , d ) μE m −2 s −1 of light and a controlled atmosphere combining 2% CO 2 and 98% air ( a , c ) and or 98% N 2 ( b , d ) to test phototrophic growth. ( e ) Cells were plated on acetate medium as heterotrophic growth control at very low light fluences (1 μE m −2 s −1 ). Full size image The light-induced oxidation of pre-reduced b l What mechanism underlies the unexpected finding that, despite its inactivated Q-cycle, the QiKO b 6 f complex sustains a flux compatible with photosynthetic growth? In the mechanistic framework of the Q-cycle, the oxidation of a quinol at the Q o site relies on the bifurcated electron transfer to the oxidized Fe 2 S 2 cluster of the Rieske subunit and to the oxidized b l haem. In the wild type, b l is quickly reoxidized by the b h haem, and thus made available as an electron acceptor for the next quinol oxidation. Consequently, in Q i KO , the long-lived reduction of the b l haem ( Fig. 3a , black trace) should only allow a single turnover of the Q o site and not a steady flux as observed here. We thus studied in vivo the function of the Q o site in conditions where a significant fraction of the b l haem was reduced ( ∼ 60%, Fig. 3a , red trace) prior to the light activation of the complex. As a fraction of b l haem was pre-reduced, the relative amplitude of the flash-induced reduction phase was smaller than that under oxidizing conditions. Saliently, we observed a net oxidation of a b haem that developed with a ∼ 250 ms half-time. The Q i site being knocked out, this net oxidation of a b haem was not electrogenic ( Fig. 4 , red trace). It must thus reflect the electron transfer from the reduced b haem to an electron acceptor produced by the light-induced injection of an oxidizing equivalent, or hole, in the high-potential chain. In principle, this hole may be borne by cytochrome f , the Fe 2 S 2 cluster or the semiquinone produced at the Q o site. The oxidized cytochrome f can be excluded as it is separated from b l by too large a distance (more than 30 Å) to allow electron transfer in a few hundred ms (ref. 17 ). The edge-to-edge distance between b l and the Fe 2 S 2 cluster ( ∼ 23 Å) is compatible with such an electron-transfer rate. However, 2-iodo-2′,4′,4′-trinitro-3-methyl-6-isopropyl diphenyl ether (DNP-INT), specifically inhibiting quinol access to the Q o site while permitting Fe 2 S 2 head domain movement ( Supplementary Fig. S4 ), prevented b l oxidation ( Supplementary Fig. S5 ). The semiquinone thus stands as the most likely candidate ( Fig. 6 ). 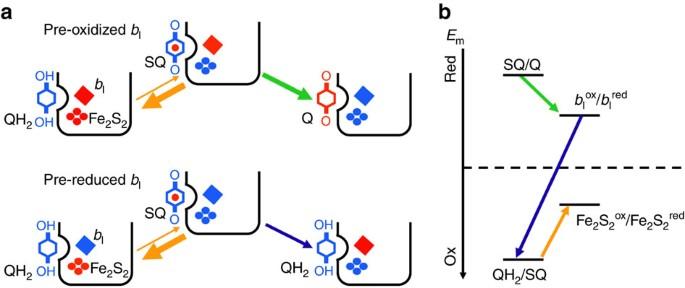Figure 6: Proposed mechanism for the turnover of the Qosite inQiKO. (a) Sequence of electron-transfer reactions depending on redox state ofbl: blue, reduced and red, oxidized. For simplicity, the semiquinone is depicted as being fully deprotonated. (b) Relative midpoint potential of the different redox couples. The arrows start from the redox couple, which provides the electron donor and point towards the redox couple providing the electron acceptor. The thicker the arrow, the larger the rate of the corresponding reaction. Figure 6: Proposed mechanism for the turnover of the Q o site in Q i KO . ( a ) Sequence of electron-transfer reactions depending on redox state of b l : blue, reduced and red, oxidized. For simplicity, the semiquinone is depicted as being fully deprotonated. ( b ) Relative midpoint potential of the different redox couples. The arrows start from the redox couple, which provides the electron donor and point towards the redox couple providing the electron acceptor. The thicker the arrow, the larger the rate of the corresponding reaction. Full size image The dual role of the semiquinone As depicted in Figure 6 , the oxidation of the quinol by the Fe 2 S 2 cluster is thought to be endergonic [18] , [19] . Recently, Zhang et al . [18] located the midpoint potential of the quinol/semiquinone couple 200 mV above that of the Fe 2 S 2 (at pH 9.0). This makes the equilibrium constant of the forward electron transfer from the quinol to the Fe 2 S 2 cluster much lower than 1 [18] , [19] . Consequently, the concentration of the reactive semiquinone is kept extremely low (see ref. 20 ) and has remained undetectable under functional conditions [21] or barely detectable (0.1–10%) under extreme ones [18] , [19] . Notably, in a cytochrome bc 1 mutant lacking the b l haem, that is, under even harsher conditions than those described here, the semiquinone has kept elusive [11] . In most of the currently considered scenarios, even though they may cover different mechanistic details, the formation of the semiquinone resulting from the oxidation of the quinol by the Fe 2 S 2 is strongly uphill in energy and is thus pulled forward by the depletion of its semiquinone product through the subsequent downhill electron transfer to the b l haem [18] , [19] , [22] . As a strong support to this mechanistic scenario, changing the driving force for quinol oxidation by changing the redox properties of the Fe 2 S 2 cluster results in linear changes in the activation energy of the Q-cycle with a slope near unity [23] . In this sequential scenario (see ref. 22 ), the injection of an electron into the high-potential chain is effectively driven by the second step, that is, the consumption of the semiquinone, and both reactions are concurrent [18] , [22] , [24] . Importantly, this behaviour is not restricted to the regular function of the Q o site but it also holds when, as we propose, the consumption of the semiquinone involves its reduction by the pre-reduced b l haem. We found accordingly that, the injection of an electron into the high-potential chain, as probed by the redox changes of cytochrome f , paralleled in time the redox changes of the b l haem irrespective of the redox poise, or, in other words, was concomitant with the redox changes of the b l haem ( Fig. 3b ). Altogether these findings show that a pre-reduced haem b l hampers, but does not preclude, the injection of an electron in the high-potential chain, that is, the quinol-plastocyanin oxidoreductase activity. A parsimonious mechanistic model accounting for these observations is a ping-pong play in which the semiquinone and the b l haem act, one after the other, as the electron donor and electron acceptor ( Fig. 6 ). This mechanism relies on the dual properties of the semiquinone species, which can act either as an electron-acceptor-yielding quinol or as an electron-donor-yielding quinone. In the currently accepted energy landscape of the bc 1 and b 6 f complexes, the semiquinone is a much stronger electron acceptor than the quinone [18] , [21] , [22] , [24] and can thus, on thermodynamic grounds, readily oxidize the b l haem to form the quinol species ( Fig. 6b ). Notably, it is yet a sluggish process with an overall rate (4 s −1 ) being several orders of magnitude slower than the theoretically predicted rate (10 6 s −1 ) [20] , [25] . It is thus kinetically limited, bringing experimental supports to a hypothesized gating mechanism (see refs 19 , 20 , 25 , 26 , 27 ). Interestingly, the overall electron-transfer flux sustained by the Q i KO b 6 f is similar to that found with the antimycin-inhibited cytochrome bc 1 [28] , [29] or the homodimer H212N bc 1 [10] , [30] . This suggests that the mechanism proposed here may also apply to the bc 1 complex, as considered in refs 28 , 29 as one among other possible scenarios. As any energy-converting enzymes, cytochrome bc 1 and b 6 f are prone to undergo short circuits in their reaction pathways. Although expected on thermodynamic grounds, appropriate mechanistic control can relegate these to extremely slow processes and thus make them negligible with regard to their yield. In keeping with this framework, we propose that a short-circuit reaction between the reduced b l and a semiquinone may occur, but that its rate would make it a poor competitor with the forward-productive electron-transfer reactions. Yet, under conditions inactivating the redox loop, the occurrence of such short circuit would provide an 'emergency exit' pathway bypassing the Q-cycle and making it dispensable. It would thereby rescue its quinol-plastocyanin oxidoreductase activity and thus the function of the entire photosynthetic chain. As mentioned above, the finding that the Q-cycle is dispensable from a mechanistic point of view also applies to the bc 1 complex, as such complex with an inhibited Q i site can sustain an overall electron-transfer flux [11] , [28] , [29] , [30] . However, it is also dispensable from an energetic standpoint in the oxygenic photosynthetic chain, whereas similar mutants of the bc 1 complex from photosynthetic purple bacteria forbid photosynthetic growth. A rationale behind this physiological difference may lie in the relative contribution of the two complexes to their respective energy-converting chain. With a fully active Q-cycle, the ratio of H + transferred across the membrane per electron transferred through the high potential chain increases from 1 to 2. The total H + /e − ratio being 2 in the photosynthetic chain of purple bacteria and 3 in the oxygenic photosynthetic chain (see Supplementary Fig. S1 ), inactivating the low-potential chain and its associated H + transfer impacts 'only' a third of the H + /e − in the latter case and up to 50% in the former. In addition, whereas the photosynthetic chain of purple bacteria promotes a cyclic electron transfer, the oxygenic photosynthetic chain allows the linear electron transfer from water to NADP + . As the mechanism we propose preserves linear electron transfer, at least partially, the impaired photosynthetic chain still yields oxygen and reducing power that can fuel the respiratory chain and thereby compensate the decreased production of ATP resulting from the inactivation of the Q-cycle and meet the requirement of the Benson–Calvin cycle in terms of ATP and reduced nicotinamide adenine dinucleotide phosphate (NADPH). To conclude, the present data show that, as in the bc 1 complex case, a disabled Q i site does not completely inhibit the function of the Q o site, which can still sustain an electron-transfer flux. In addition, we show that, at odds with the bc 1 complex case, this flux is large enough to allow photosynthetic growth, thus demonstrating that, in the oxygenic photosynthetic chain, the Q-cycle is dispensable from an energetic standpoint. Strains and growth conditions The following C. reinhardtii strains were grown heterotrophically in continuous white light (5 μE m −2 s −1 ) in Tris–acetate–phosphate medium, pH 7.2 at 25 °C: wild type, deletion of chloroplast petB gene encoding cytochrome b 6 Δ petB [31] , substitution of b h haem ligand petB-H202Q [6] , [12] , His-tag addition in chloroplast petA gene encoding cytochrome f petA-CterH 6 [5] ), substitution of ATP-dependent FtsH protease arginine finger that is essential for ATPase and protease activity [13] in nuclear-encoded FtsH1 gene ftsH1-R420C [14] , and combinations isolated by sexual crosses [32] and chloroplast transformation ftsH1-R420C{petB-H202Q} ( Q i KO ), ftsH1-R420C{petA-CterH 6 } and ftsH1-R420C{petA-CterH 6 ;petB-H202Q} . Growth tests were initiated by spotting 10 5 cells of log-phase cultures onto agar plates. Plates were placed in tight-sealed chambers applying 2% CO 2 and 98% N 2 with a gas flowmeter (Aalborg) for anaerobiosis. Immunoblot analysis Cell proteins were separated on 12–18% SDS–polyacrylamide gels containing 8 M urea, electrotransferred onto polyvinylidene fluoride membranes, revealed for haem peroxidase activity by femto chemiluminescence, and immunodetected using antibodies against C. reinhardtii proteins by chemiluminescence [6] . His-tagged Q i KO strain construct Plasmid pB202QK was constructed by introducing the Eco RV– Sma I fragment of plasmid pUC-atpX-AAD bearing the aadA cassette conferring spectinomycin resistance [33] downstream and in the same orientation as the petB gene at the unique Nsi I site of plasmid pB202Q carrying the mutation petB-H202Q , and was transformed [12] in strain ftsH1-R420C{petA-CterH 6 } to generate a His-tagged Q i KO . In vitro analysis Cytochrome b 6 f complex was purified as in ref. 5 and its in vitro activity was assessed as in ref. 16 using petA-CterH 6 and ftsH1-R420C{petA-CterH 6 ;petB-H202Q} strains after proper non-specific activity subtraction. Spectroscopic analysis Electrogenicity of electron transfers and redox changes of cytochromes b and f were assessed by monitoring absorbance at 520, 546, 554, 564 and 573 nm with a JTS10 spectrophotometer (BioLogic). Cytochrome b redox changes were measured at 564 nm with a baseline drawn between 546 and 573 nm. Cytochrome f redox changes were measured at 554 nm with a baseline drawn between 546 and 573 nm and the intensity of the actinic was tuned to hit 30% photosystem I. In addition, the latter were corrected for the contribution of the electrochromic bandshift by subtracting 5% of the absorption changes measured at 520 nm. The cytochrome absorbance changes were calibrated on the basis of normalization to the cytochrome f content in the WT . Control of the redox poise Cells were dark-adapted in 20 mM Hepes, 20% Ficoll, pH 7.2. A 5-ns and 1-mJ cm −2 laser flash was used to activate light reactions. To achieve mildly reducing conditions, cells were thoroughly mixed and aerated before absorbance measurement for each wavelength probed. Cells were kept in the sample cell in the dark for a time ranging from 1 to 3 min depending on the strain used and their respiration rate. Strongly reducing conditions were obtained by adding 20 mM glucose, 2 mg ml −1 glucose oxidase to achieve anoxia, and mediators anthraquinone (−100 mV) and anthraquinone-2-sulphonate (−225 mV) at 1 μM to promote redox poising of the cells and thus b l haem reduction [34] . The sample was kept in the dark for 25 min under complete anoxia. We have checked (not shown) that the first quinone acceptor of photosystem II was fully reduced under such conditions. The time between two consecutive actinic flashes was set at 5 min, to allow the redox equilibration of the samples between flashes. To obtain a similar content of pre-reduced and pre-oxidized b haem in the Q i KO strain, the cells were first dark adapted for 25 min under complete anoxia, yielding the strongly reducing case described above, and then submitted to a series of 5 pre-illuminating flashes at 0.2 Hz. Inhibitors Two distinct Q o site inhibitors were used: tridecyl-stigmatellin and 2-iodo-2′,4′,4′-trinitro-3-methyl-6-isopropyl diphenyl ether. PSII was inhibited by 1 mM hydroxylamine and 10 μM 3-(3,4-dichlorophenyl)-1,1-dimethylurea (DCMU) to determine the PSII:PSI ratio for normalization. How to cite this article: Malnoë, A. et al . Photosynthetic growth despite a broken Q-cycle. Nat. Commun. 2:301 doi: 10.1038/ncomms1299 (2011).